Quantum fluctuations in spin-ice-like Pr2Zr2O7 Spin ice is a magnetic analog of H 2 O ice that harbors dense static disorder. Dipolar interactions between classical spins yield a frozen frustrated state with residual configurational Pauling entropy and emergent magnetic monopolar quasiparticles. Introducing quantum fluctuations is of great interest as this could melt spin ice and allow coherent propagation of monopoles. Here, we report experimental evidence for quantum dynamics of magnetic monopolar quasiparticles in a new class of spin ice based on exchange interactions, Pr 2 Zr 2 O 7 . Narrow pinch point features in otherwise diffuse elastic neutron scattering reflects adherence to a divergence-free constraint for disordered spins on long time scales. Magnetic susceptibility and specific heat data correspondingly show exponentially activated behaviors. In sharp contrast to conventional ice, however, >90% of the neutron scattering is inelastic and devoid of pinch points furnishing evidence for magnetic monopolar quantum fluctuations. Classical Ising spins with dipolar interactions on the pyrochlore lattice possess a macroscopically degenerate ensemble of ground states [1] , [2] . Satisfying the two-in two-out ice rule on each tetrahedron [3] , [4] , these states of rare-earth spins in magnets such as Dy 2 Ti 2 O 7 and Ho 2 Ti 2 O 7 are in one-to-one correspondence with the disordered configurations of protons in H 2 O ice ( Fig. 1a ). Mimicking the formation of an H 3 O + –OH − electric dipole in water ice, a spin flip from the spin ice manifold fractionalizes into a pair of emergent magnetic monopolar quasiparticles with Coulomb attraction [5] , [6] , [7] , [8] , [9] . 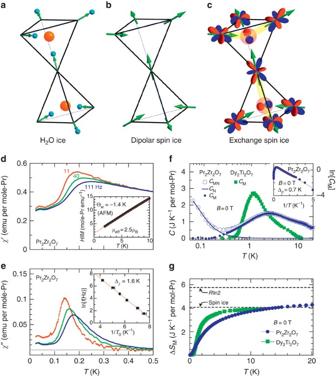Figure 1: Structures of different types of ice, and thermodynamic response of Pr2Zr2O7. (a,b,c) A fragment of the pyrochlore structure is shown to illustrate the 2-in 2-out ice rule for the configuration of proton (blue sphere) and oxygen (red sphere) sites in water ice (a), classical Ising spins (green arrows) with dipolar interaction in spin ice (b), and theD3dcrystal electric field doublet ground state wave function in exchange spin ice with superexchange interactions mediated by oxygen 2porbitals at the center of each tetrahedron (c). The signs of the 4fand 2pwave functions are denoted by red and blue colors. The light yellow belt indicates a superexchange path. (d) Real part of the AC-susceptibility (χ′). Inset: DC field divided by magnetizationH/M(T) for temperatures from 10 K to 2 K andμ0H=0.1 T. (e) Imaginary part of the AC-susceptibility (χ′′). Inset: measurement frequency versus inverse freezing temperature defined as the peak temperature for χ′′(T). The solid line denotes a fit to the Arrhenius law, which yields an activation energy Δχ=1.62(3) K. (f) Magnetic and nuclear part of the specific heatCMNfor Pr2Zr2O7after subtracting lattice and CEF contributions in zero field (open blue circle) (seeSupplementary Note 4for details). A refined estimateCM=CMN−CN(filled blue circle) was obtained by subtracting a scaled nuclear Schottky-like anomaly (solid blue line).CMfor Dy2Ti2O7, adapted from ref.2, is also shown for comparison (filled green square). Inset:CMversus 1/Ton a semi-logarithmic scale. The solid line denotes a fit to an Arrhenius law between 2 to 0.2 K, which yields an activation energy of 0.72(1) K. (g) Magnetic entropy ΔSM(filled blue circle) for Pr2Zr2O7calculated fromCM. Open green squares show ΔSMfor Dy2Ti2O7(ref.2). The dashed black lines denote the entropy for a two level system () and the spin ice entropy defined as the difference betweenand the Pauling entropy of=0.292. Figure 1: Structures of different types of ice, and thermodynamic response of Pr 2 Zr 2 O 7 . ( a , b , c ) A fragment of the pyrochlore structure is shown to illustrate the 2-in 2-out ice rule for the configuration of proton (blue sphere) and oxygen (red sphere) sites in water ice ( a ), classical Ising spins (green arrows) with dipolar interaction in spin ice ( b ), and the D 3 d crystal electric field doublet ground state wave function in exchange spin ice with superexchange interactions mediated by oxygen 2 p orbitals at the center of each tetrahedron ( c ). The signs of the 4 f and 2 p wave functions are denoted by red and blue colors. The light yellow belt indicates a superexchange path. ( d ) Real part of the AC-susceptibility ( χ ′). Inset: DC field divided by magnetization H / M ( T ) for temperatures from 10 K to 2 K and μ 0 H =0.1 T. ( e ) Imaginary part of the AC-susceptibility (χ′′). Inset: measurement frequency versus inverse freezing temperature defined as the peak temperature for χ′′( T ). The solid line denotes a fit to the Arrhenius law, which yields an activation energy Δ χ =1.62(3) K. ( f ) Magnetic and nuclear part of the specific heat C MN for Pr 2 Zr 2 O 7 after subtracting lattice and CEF contributions in zero field (open blue circle) (see Supplementary Note 4 for details). A refined estimate C M = C MN − C N (filled blue circle) was obtained by subtracting a scaled nuclear Schottky-like anomaly (solid blue line). C M for Dy 2 Ti 2 O 7 , adapted from ref. 2 , is also shown for comparison (filled green square). Inset: C M versus 1/ T on a semi-logarithmic scale. The solid line denotes a fit to an Arrhenius law between 2 to 0.2 K, which yields an activation energy of 0.72(1) K. ( g ) Magnetic entropy Δ S M (filled blue circle) for Pr 2 Zr 2 O 7 calculated from C M . Open green squares show Δ S M for Dy 2 Ti 2 O 7 (ref. 2 ). The dashed black lines denote the entropy for a two level system ( ) and the spin ice entropy defined as the difference between and the Pauling entropy of =0.292 . Full size image In classical spin ice, monopole dynamics is diffusive—only activated thermally or by external magnetic field [5] , [6] , [10] as solitons in semiclassical spin chains [11] . The classical nature of Ising spins precludes attainment of thermal equilibrium at temperatures ( T ) below the effective nearest neighbor energy scale J ff . Quantum fluctuations enhance dynamics and might allow coherent propagation of magnetic charge [12] , [13] , [14] , [15] , much as spinons in one-dimensional quantum magnets [16] . Contrary to H 2 O ice, pyrochlore-based rare-earth spin systems [17] provide excellent opportunities to explore quantum effects in ice. Quantum fluctuations were theoretically proposed as the origin of a putative spin liquid in Tb 2 Ti 2 O 7 (ref. 18 ). More recently, experimental work on Pr 2 Ir 2 O 7 shows the possibility of a chiral spin liquid phase when quantum fluctuations melt spin ice [19] , [20] . Strong spin fluctuations were observed for Pr 2 Sn 2 O 7 (ref. 21 ) and Yb 2 Ti 2 O 7 (refs 22 , 23 , 24 , 25 ), which have spin ice correlations. There, superexchange interactions for the smaller moment Pr 3+ and Yb 3+ systems are much stronger than dipolar interactions; so, the materials are referred to as exchange(-based) spin ice ( Fig. 1c ) [24] , [26] . In this class of spin ice, the two-in two-out states should no longer be static, but dynamic—described by a quantum superposition of the spin ice manifold. Here, we report the experimental observation of spin ice correlations and quantum dynamics in Pr 2 Zr 2 O 7 . Magnetic properties Thermomagnetic measurements on Pr 2 Zr 2 O 7 provide key insights particularly when compared with the classical spin ice compounds ( Fig. 1 ). We have succeeded in growing high-quality single crystals, which are stoichiometric to the 1–2% level, as determined by chemical analyses and single crystal synchrotron X-ray diffraction measurements ( Supplementary Figures S1 and S2 , Supplementary Tables S1 and S2 , and Supplementary Note 1 ). The temperature-dependence of the inverse susceptibility of single crystalline Pr 2 Zr 2 O 7 exhibits Curie–Weiss behavior for T < 10 K with an effective moment μ eff =2.5(1) μ B ( Fig. 1d , inset) that is four times smaller than for dipolar spin ice Dy 2 Ti 2 O 7 where μ eff =10 μ B . Correspondingly, Pr 2 Zr 2 O 7 displays an antiferromagnetic Weiss temperature Θ W =−1.4(1) K compared with the ferromagnetic Θ W ≈ +0.5 K for dipolar Dy 2 Ti 2 O 7 (ref. 2 ). While no anomaly indicating long-range ordering was found down to 20 mK, AC-χ( T ) exhibits a frequency-dependent peak at T 0 ( f ), which is the onset temperature for dynamics at the frequency, f ( Fig. 1d ). The data for T 0 ( f ) ( Fig. 1e , inset) are consistent with thermal activation over at least three decades. For classical spin ice, the corresponding activation energy Δ χ =1.62(3) K, is the spin flip energy, 2 J ff , from the ice manifold. Though the activation energies are similar, the limiting (attempt) frequency f 0 ~1 MHz for Pr 2 Zr 2 O 7 is three orders of magnitude larger than for Dy 2 Ti 2 O 7 (refs 10 , 27 ). Moreover, upon cooling to the lowest T , the real part of AC-χ( T ) approaches 50% of the peak height while it vanishes for Dy 2 Ti 2 O 7 (refs 27 , 28 ). These indicators of enhanced fluctuations at low temperatures are consistent with general expectations for a quantum spin system. Crystal electric field To determine the crystal electric field (CEF) scheme, we used inelastic neutron scattering and found five magnetic excitations at energy transfers 9.5 meV, 57.1 meV, 81.9 meV, 93.2 meV and 109 meV ( Fig. 2 ). Simultaneous fitting of a crystal field model to neutron and magnetic susceptibility data ( Fig. 2 ) shows the ground state is a magnetic doublet with (111) Ising anisotropy, as in classical spin ice systems [1] ( Supplementary Tables S3, S4 , and Supplementary Note 2 ). This is, however, not a Kramers doublet; so, although the specific heat data ( Fig. 1f ) show there is no conventional Jahn-Teller transition, magneto-elastic effects may have an important role in Pr 2 Zr 2 O 7 . 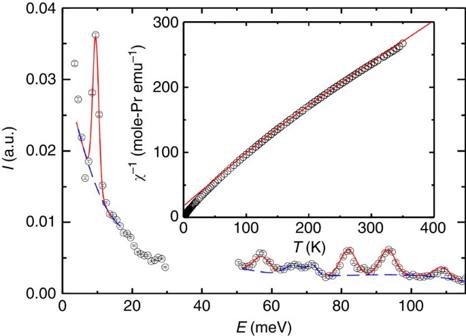Figure 2: Crystal electric field analysis of inelastic neutron scattering and susceptibility. Main panel: magnetic excitation spectrum obtained by combiningT=7.8 K data for two incident beam energies:Ei=40 meV andEi=120 meV. The blue dashed line denotes fitted polynomial backgrounds. The red solid line is the calculated best fit. Inset: temperature dependence of the inverse magnetic susceptibility. The red solid line in the inset was calculated using the same crystal field parameters as used to account for the neutron scattering data (Supplementary Tables S3 and S4). Details are provided in theSupplementary Note 2. Figure 2: Crystal electric field analysis of inelastic neutron scattering and susceptibility. Main panel: magnetic excitation spectrum obtained by combining T =7.8 K data for two incident beam energies: E i =40 meV and E i =120 meV. The blue dashed line denotes fitted polynomial backgrounds. The red solid line is the calculated best fit. Inset: temperature dependence of the inverse magnetic susceptibility. The red solid line in the inset was calculated using the same crystal field parameters as used to account for the neutron scattering data ( Supplementary Tables S3 and S4 ). Details are provided in the Supplementary Note 2 . Full size image Elastic and inelastic neutron scattering Low-energy transfer neutron-scattering data provide a direct view of dynamics in the spin ice state. A 40 mm × 20 mm 2 cylindrical single crystal was used to achieve sufficient magnetic scattering intensity from the relatively small Pr 3+ moments. Nominally elastic magnetic scattering covering broad regions of momentum space develops upon cooling from 22 K to 0.1 K, indicating short-range quasi-static spin correlations ( Fig. 3b ). Sharp pinch point features near (111) and particularly (002), bear evidence of a divergence-free two-in two-out spin configuration on each tetrahedron [9] , [25] , [29] , [30] . Indeed, the elastic Q -map resembles a classical Monte Carlo simulation for an exchange-only model [9] , [29] , which indicates dominant ferromagnetic superexchange interactions in Pr 2 Zr 2 O 7 . Θ W is, however, negative and this suggests—consistent with recent theoretical predictions [31] , [32] —the exchange Hamiltonian includes antiferromagnetic transverse terms that induce quantum dynamics. Though the ground state doublet is Jahn–Teller active, the observed scattering does not resemble that predicted for a model where the local three fold axis is broken [30] . 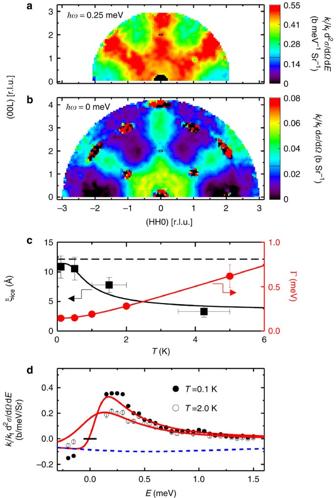Figure 3: Spin ice correlations and quantum dynamics probed with elastic and inelastic neutron scattering. (a) InelasticQ-map with energy transfer of 0.25 meV obtained after subtracting the corresponding data at 15 K as background. The broad diffuse scattering pattern carries the symmetry of the crystal but cannot be associated with phonon scattering, which is concentrated around strong nuclear Bragg peaks at low energies. Instead we associate it with inelastic magnetic scattering. The fact that the scattering is wave vector dependent further links it to inter-site quantum spin dynamics. (b) ElasticQ-map with pinch points at (002), (111), and (). By subtracting 22 K data from 0.1 K data to cancel elastic nuclear scattering processes at Bragg peaks, we obtain quasi-static spin correlations on the time scale ofτ=/δE=2 ps. The black ellipses at (002) in (a) and (b) indicate the full width at half maximum instrumental resolution. (c) Temperature-dependence of the spin ice correlation lengthξice(left) and the relaxation rate Γ (right). The black solid line denoteswith the activation energy fixed at the value of Δχ=1.62(3) K. The red solid line shows, whereC=1.4(2). The black horizontal dashed line indicates the mean distance between 1% of the Pr sites, which according to synchrotron X-ray analysis are occupied by Zr (Supplementary Figure S2andSupplementary Note 1). (d) Inelastic neutron scattering (INS) spectra atQ=(003) andT=0.1 K (solid circle) and 2.0 K (open circle) after subtraction of INS data obtained at the sameQbut at the elevated temperature of 15 K. A correction to the monitor rate was applied to account for order contamination in the unfiltered incident beam. The fitting curve and the corresponding background resulting from subtraction of magnetic scattering atT=15 K to derive Γ are shown by red solid and blue dashed curves, respectively. The details of the analysis are described inSupplementary Note 3. The error bars reflect one s.d. counting statistics. When error bars are not visible they are smaller than the symbol size. Figure 3: Spin ice correlations and quantum dynamics probed with elastic and inelastic neutron scattering. ( a ) Inelastic Q -map with energy transfer of 0.25 meV obtained after subtracting the corresponding data at 15 K as background. The broad diffuse scattering pattern carries the symmetry of the crystal but cannot be associated with phonon scattering, which is concentrated around strong nuclear Bragg peaks at low energies. Instead we associate it with inelastic magnetic scattering. The fact that the scattering is wave vector dependent further links it to inter-site quantum spin dynamics. ( b ) Elastic Q -map with pinch points at (002), (111), and ( ). By subtracting 22 K data from 0.1 K data to cancel elastic nuclear scattering processes at Bragg peaks, we obtain quasi-static spin correlations on the time scale of τ =/δ E =2 ps. The black ellipses at (002) in ( a ) and ( b ) indicate the full width at half maximum instrumental resolution. ( c ) Temperature-dependence of the spin ice correlation length ξ ice (left) and the relaxation rate Γ (right). The black solid line denotes with the activation energy fixed at the value of Δ χ =1.62(3) K. The red solid line shows , where C =1.4(2). The black horizontal dashed line indicates the mean distance between 1% of the Pr sites, which according to synchrotron X-ray analysis are occupied by Zr ( Supplementary Figure S2 and Supplementary Note 1 ). ( d ) Inelastic neutron scattering (INS) spectra at Q =(003) and T =0.1 K (solid circle) and 2.0 K (open circle) after subtraction of INS data obtained at the same Q but at the elevated temperature of 15 K. A correction to the monitor rate was applied to account for order contamination in the unfiltered incident beam. The fitting curve and the corresponding background resulting from subtraction of magnetic scattering at T =15 K to derive Γ are shown by red solid and blue dashed curves, respectively. The details of the analysis are described in Supplementary Note 3 . The error bars reflect one s.d. counting statistics. When error bars are not visible they are smaller than the symbol size. Full size image The transverse width of the pinch points in elastic neutron scattering is a measure of the density of Pr tetrahedra that violate the ice rule [7] , hence the monopole density. To determine this density, we measured the pattern of elastic magnetic neutron scattering near the Q =(002) pinch point with a high-resolution configuration. Two configurations of the MACS instrument were used for this experiment. For rapid high statistical mapping of Q -dependent scattering, we used a fixed final neutron energy E f =5 meV. The corresponding measured energy resolution δ E =0.38 meV and the calculated principal axes of the Q resolution near (002) are δ Q 1 =0.093 Å −1 and δ Q 2 =0.041 Å −1 . For high-resolution measurements, we used E f =2.7 meV, where δ E =0.12 meV, δ Q 1 =0.093 Å −1 , δ Q 2 =0.025 Å −1 , and the incoherent elastic count rate is reduced by a factor 5. The pinch point width was extracted by fitting the following phenomenological model of scattering to two-dimensional intensity maps in the (HHL) reciprocal lattice plane [7] , [9] (see Supplementary Note 3 for details): Both the quasi-static (τ>/δ E =6 ps) total moment S (0), and the spin ice correlation length ξ ice increase on cooling ( Fig. 3c and Supplementary Figure S3 ). The low T limit, ξ 0 , indicates a quasi-static monopole density of 1.2%. This can be compared with the ~1% concentration of Zr on Pr sites determined by single crystal synchrotron X-ray diffraction ( Supplementary Figure S2 and Supplementary Note 1 ). The fitting function, , (black solid line, Fig. 3c ) describes the data well with the activation energy fixed at the value of Δ χ =1.6 K extracted from AC-χ( T ) data ( Fig. 1e , inset). The wave vector map of inelastic scattering at ω=0.25 meV and T =0.1 K is shown in Fig. 3a . As ħ ω >> k B T ~0.01 meV, the inelastic scattering is evidence for quantum spin dynamics and the frequency scale of ν = ω/2π =60 GHz sets it apart from the thermally activated spin dynamics probed by AC susceptibility measurements on the kHz frequency scale. While the overall pattern resembles the nominally elastic scattering ( Fig. 3b ), the pinch points have vanished. Excited states thus differ from the ground state by the appearance of tetrahedra that violate the ice rule or in other words by the presence of magnetic monopoles. Combined, the elastic scattering that does show pinch points and the inelastic scattering that does not, constitute experimental evidence for magnetic monopoles with quantum dynamics. By normalizing the intensity data ( Supplementary Note 3 and Supplementary Figure S3 ), we find that such inelastic scattering accounts for >90% of the magnetic scattering cross section of the low-energy CEF doublet at T =0.1 K. This shows magnetism in Pr 2 Zr 2 O 7 is dominated by quantum fluctuations. To characterize the monopole fluctuation spectrum, we carried out constant Q =(003) scans at various T s, subtracting T =15 K data as a background ( Fig. 3d ). The low T spectrum places an upper limit of Δ E =0.2 meV on any excitation gap. Upon heating the spectrum broadens and to quantify this effect, we fitted the T -difference data to the scattering associated with a single imaginary pole response, χ(ω)=χ 0 Γ/(Γ− iω ), accounting for the background subtraction with a consistent T =15 K relaxation rate as detailed in Supplementary Note 3 . Figure 3c shows the T -dependence of the relaxation rate, Γ. At high temperatures, Γ might be interpreted as a monopole relaxation rate. The red solid line shows , where C =1.4(2). The crossover to linearity and thus ω / T scaling is evidence of a regime for T > J ff , where T is the only relevant energy scale. In the low T limit, Γ~0.17 meV is similar to the spin flip energy 2 J ff =Δ χ ~1.6 K inferred from AC- χ ( T ). The observation of a broad spectrum rather than a sharp spin flip mode indicates monopole quantum dynamics [12] , [14] , [15] . A possible low-energy regime of photons predicted for a U (1) spin liquid [12] , [14] , [15] , however, cannot be resolved in the present neutron scattering experiment. Heat capacity Complementary information about the excitation spectrum is provided by specific heat measurements ( Fig. 1f ) (see Supplementary Note 4 for details). After subtraction of the lattice and CEF contributions, the temperature-dependence of the magnetic and nuclear-specific heat C MN ( T ) does not exhibit sharp features that would result from long-range ordering or a conventional Jahn–Teller transition. Instead, a broad peak at T ~2 K ~Δ χ =2 J ff ~1.6 K ( Fig. 1f ) can be associated with the proliferation of thermally activated monopole pairs. While the position of the peak is similar to that for Dy 2 Ti 2 O 7 , the greater width is consistent with the broad spectrum of inelastic neutron scattering and monopole quantum dynamics in Pr 2 Zr 2 O 7 . The upturn in C MN ( T ) below ~200 mK provides valuable information about electronic dynamics on the nuclear spin time scale. A fully frozen state of ~3.0 μ B Pr moments would generate a nuclear Schottky peak at ~0.17 K with a height of ~7 J mol −1 K −1 , which is inconsistent with the data. Instead, as shown in Fig. 1f , the upturn can be fitted by C N ( T )= f × C Sch ( T ), where C Sch ( T ) is a full expression of nuclear Schottky-specific heat with a hyperfine coupled Pr moment and f =0.37 is a dimension-less factor representing the fraction of Pr sites with the dipole moment ( Supplementary Note 4 ). The corresponding elastic neutron scattering cross section barn is not inconsistent with the low T magnetic scattering cross section of 0.02 barn within the 0.1 meV energy resolution of the experiment ( Supplementary Figure S3 ). Here g J =4/5, r 0 =−0.54 × 10 −12 cm and =2/3 is the spherical average of the polarization factor for Ising spins. The reduced frozen moment indicates strong quantum fluctuations [33] as does the large value of the real part of the AC-susceptibility χ′( T ) in the low T limit ( Fig. 1d ). The apparent inhomogeneity indicated by f =0.37<1 suggests the weak frozen moment could be an extrinsic feature resulting from extreme sensitivity to chemical inhomogeneity. Assigning in this way the low T upturn to nuclear spins, the electronic entropy obtained by integrating C M / T =( C MN − C N )/ T up to 20 K is , which is close to the value of for classical ice [2] , [4] ( Fig. 1f ) and inconsistent with a full static Jahn–Teller distortion [34] . The inferred zero-field magnetic component C M shows a decade of activated T -dependence between 2 K and 0.2 K ( Fig. 1f , inset). The corresponding activation energy of Δ C =0.72(1) K is approximately half of that associated with AC-susceptibility data Δ χ =1.62(3) K. Note, however, that the above interpretation is not unique and we cannot exclude the possibility that the low T upturn in C MN ( T ) involves both nuclear and electronic spin entropy. From the multiple streams of distinct but consistent data presented, the following key characteristics of Pr 2 Zr 2 O 7 emerge. (1) Strong quantum fluctuations: At T =0.1 K, >90% of the magnetic scattering cross section is inelastic, the attempt frequency associated with the activated AC susceptibility is three orders of magnitude larger than for classical spin ice, and the nuclear Schottky anomaly is suppressed below that for a classical frozen state both in terms of moment density and magnitude. (2) Weak static correlations: while exponentially activated specific heat and AC susceptibility data, elastic magnetic neutron scattering, and the nuclear Schottky anomaly consistently indicate some spin-freezing, this could be an extrinsic consequence of weak chemical inhomogeneities. (3) Spin-ice-like correlations at long times: the wave vector dependence of the lowest energy scattering detected features pinch points, the width of which is consistent with the inferred chemical defect density. While further experimental work is required to fully determine the ground state of Pr 2 Zr 2 O 7 in the clean limit, it is safe to say that it features quantum fluctuations of magnetic monopoles and is unlike any previously documented in an insulating crystalline magnet. The interplay between monopolar quantum dynamics and itinerant electrons may have an important role in the isostructural Kondo lattice system Pr 2 Ir 2 O 7 (refs 19 , 20 ). Sample preparation Single crystalline samples of Pr 2 Zr 2 O 7 were grown by a floating zone method [35] . The orientation of each crystals was established by X-ray Laue diffraction. Energy dispersive X-ray analysis found no impurity phases and determined the Pr/Zr ratio to be 0.94(3). Synchrotron X-ray diffraction measurements were performed at SPring-8. Structure analysis, detailed in Supplementary Note 1 , confirmed the pyrochlore crystal structure with symmetry. The crystal structure information is provided in Supplementary Tables S1 and S2 . Further analysis of the diffraction data indicates no significant site mixing beyond the detection limit, but Pr-deficiency at the ~1% level ( Supplementary Figures S1, S2 , and Supplementary Note 1 ). A single crystal of the non-magnetic analog La 2 Zr 2 O 7 was also grown by a floating zone method, and used to approximate the lattice specific heat of Pr 2 Zr 2 O 7 . Measurement of magnetic properties The temperature-dependence of the DC magnetization at a field of 1000 Oe above 2 K was measured using a commercial SQUID magnetometer. The temperature dependence of the AC susceptibility at an excitation field of 0.3 Oe below 5 K was measured down to 20 mK in a dilution refrigerator through a mutual inductance method. For both measurements, the field was applied along the [111] direction. The AC susceptibility data sets were scaled to data collected at 1000 Oe for temperatures above 2 K. For all data, a demagnetization correction was made with a demagnetization factor N =0.2 obtained by approximating the sample shape as a rectangular prism [36] . The temperature-dependence of the specific heat was measured by a thermal relaxation method down to 0.07 K. A thin platelet single crystal with a (111) surface normal was used to achieve good thermal contact. Details regarding the analysis of specific heat date are provided in Supplementary Note 4 . Neutron scattering measurements Neutron scattering measurements were carried out on a 0.8 cm 3 single crystal sample using the MACS spectrometer at the NIST Center for Neutron Research for energy transfer below 2 meV and the ARCS spectrometer at the Spallation Neutron Source, Oak Ridge National Laboratories for energy transfer up to 120 meV. The detailed methods of data collection and analysis employed for ARCS and MACS are described in Supplementary Notes 2 and 3 respectively. How to cite this article: Kimura, K. et al . Quantum fluctuations in spin-ice-like Pr 2 Zr 2 O 7 . Nat. Commun. 4:1934 doi: 10.1038/ncomms2914 (2013).